Interference and holography with femtosecond laser pulses of different colours Interferometry and holography are two domains that are based on observation and recording of interference fringes from two light beams. While the aim of the first technique is to reveal and map the phase difference of two wave fronts, the main task of the second technique is to reconstruct one of the two recording waves via diffraction of the other wave from the recorded fringe pattern (hologram). To create fringes, mutually coherent waves from the same laser are commonly used. It is shown here that fringes can be observed and holograms can be recorded with ultrashort, sub-picosecond pulses even of different colour, generated in our experiment with two parametric amplifiers seeded, both by the same mode-locked Ti-sapphire laser. The appearance of permanent and transient gratings is confirmed by recording of an image-bearing hologram, by observation of two-beam coupling gain in a pump–probe experiment and by frequency conversion in Raman–Nath self-diffraction from a moving grating. The idea of wavefront recording and reconstruction, known today as holography, was formulated by Gabor [1] . His proof-of-principle experiment was done with the light of a high pressure mercury lamp; it was necessary, however, to wait more than a decade for the invention of lasers to ensure holographic recording with really high quality of image reconstruction. A source of coherent radiation is necessary to form the interference pattern of the object wave and reference wave, that could be replicated in the recording material as a hologram. The important requirement to the light source is also its sufficiently large coherence length to ensure high enough contrast of fringes formed by different components of the object wave with the reference wave. Thus, it is universally accepted now that to record a hologram, both waves—object and reference—should be generated from the same laser, which emits, preferably, a single longitudinal TEM 00 mode. In this article, we report on experiments aiming the holographic grating recording with two laser sources that generate, in addition, light with considerably different optical frequencies, more precisely blue and green light. The success of this counterintuitive experiment is ensured by using ultrashort, ≈100 fs pulses from two different optical parametric amplifiers (OPAs). In our particular experiment, the fringes formed by a blue beam with a green one are moving with a speed only three times smaller than light velocity. With 100 fs pulses, however, the displacement of the fringe pattern as a whole is less or comparable with one fringe spacing and the fringe contrast averaged over the pulse duration is still quite high. The field of femtosecond holography is already well-established today by the successful demonstration of static holograms recording (see, for example, refs 2 , 3 , 4 , 5 ). So far, the recording was performed in a traditional way by beams from the same femtosecond laser, the spectral content of the two recording beams being identical. Also, starting from papers of Froehly et al . [6] the so called ‘spectral holography’ [6] , [7] , [8] (and later ‘spectral nonlinear optics’ [9] ) was used for recording, reconstruction and processing of temporal envelopes of the short pulses. In a series of papers initiated by a publication of Buse et al . [10] , light with the wavelength other than that necessary for grating recording was used to improve the holographic sensitivity of the medium (some researchers called it ‘two-colour holography’). In all above papers, as also in similarly oriented other papers, the recording of permanent holographic gratings by beams with considerably different frequencies was never considered. Our interest in grating recording with beams of different colour is motivated by its possible impact on the field of ultrafast optics, where the interaction of two or more ultrashort laser pulses within an optical medium is a common situation. The researchers face it in fundamental studies and in different applications, from frequency conversion to sensitive measurements of nonlinear constants of optical materials used in this domain. At present, the absolute majority of papers that treat nonlinear interaction of two short pulses with different photon energies focus on a coupling that depends on the integral intensities, I pu and I pr (subscripts pu and pr mark pump and probe pulses, respectively). These intensities are different for different frequencies ω , depend on time t and propagation coordinate z . However, the interference of the pulse fields, that is, the small scale variations of total intensity in transverse direction x is disregarded in the case of different pulse frequencies. This can result in unexpected experimental observations or lead to misinterpretation of the obtained data sets, because the self-diffraction from the grating, which might be recorded by these fringes, brings by itself an additional direct beam coupling. The unusual result of our pump–probe experiments with LiNbO 3 crystal described below, in the beginning of the next section, serves as a representative example. An example of possible application of the considered phenomenon, the frequency (up and down) conversion, is demonstrated, which is because of the Raman–Nath diffraction from the the moving grating recorded by pulses of different colours. Manifestation of self-diffraction in pump–probe experiments When trying to clarify the formation dynamics of small electron (or hole) polarons [11] in LiNbO 3 , the normalized probe pulse transmission Δ T / T was measured in a range −500 fs≤Δ t ≤1,000 fs of the probe pulse delay times. These measurements have been performed within a broad spectral range of probe wavelength variation, 400 nm≤ λ ≤900 nm, with the intention to cover spectral manifestations of the small polarons, the pump wavelength being fixed at 490 nm. 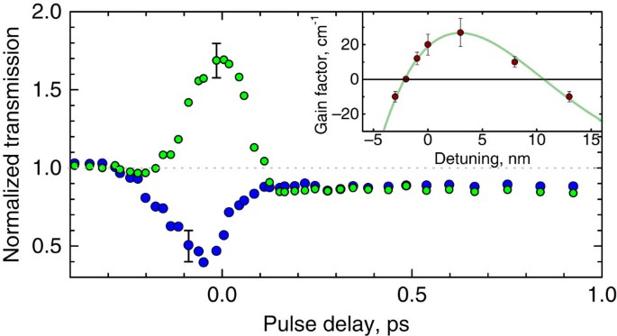Figure 1: Pump–probe experiment with LiNbO3. The probe beam transmission versus time delay of the probe pulse with respect to the pump pulse. The wavelengths of the probe pulse are 485 nm and 493 nm for blue and green dots, respectively, the pump wavelength is≃490 nm. The inset shows the detuning dependence of the net gain factor (amplification minus absorption) for probe and pump pulses matched in time. Figure 1 shows the normalized probe pulse transmission Δ T / T as a function of the probe pulse delay time Δ t with respect to the pump pulse. For large wavelength detunings (much larger than the full-width at half maximum (FWHM) of the pulse spectral content ≈5 nm) the measured dependence shows a well-known dip at Δ t =0, which is due to the two-photon absorption (blue data dots, see, for example, ref. 12 ). The unusual and intuitively unexpected feature is the observation of a probe pulse enhancement, instead of depletion, within a considerably large wavelength interval in the vicinity of total degeneracy. The amplification of the probe pulse with the wavelength 493 nm is shown in Fig. 1 by green dots. Figure 1: Pump–probe experiment with LiNbO 3 . The probe beam transmission versus time delay of the probe pulse with respect to the pump pulse. The wavelengths of the probe pulse are 485 nm and 493 nm for blue and green dots, respectively, the pump wavelength is ≃ 490 nm. The inset shows the detuning dependence of the net gain factor (amplification minus absorption) for probe and pump pulses matched in time. Full size image The inset to the Fig. 1 gives the wavelength detuning dependence of a formally introduced exponential gain factor γ =(1/ ℓ )ln T ( ℓ is the sample thickness). It suggests that the gain becomes large enough to overcome the two-photon absorption within the detunings range of −3 nm≤Δ λ ≤+8 nm. The processes of optical parametric amplification can be excluded in explanation of these findings, instead, the probe amplification by means of self-diffraction from a grating recorded by the pump and probe beams [13] , [14] seems to be very probable. Several facts support this hypothesis, among them, the absence of gain in the case of cross-polarized pump and probe pulses and characteristic changes in the spectra of the amplified probe, with a signature of the pump pulse spectrum. Thus, the inertial grating recording with pulses that differ in wavelengths about 5 nm or more must be considered. The question arises, is such a recording possible at all and, if yes, how large the allowed frequency detuning can be. These fundamental questions are addressed qualitatively and analytically below. Qualitative considerations and estimates After seminal publication [1] , it became clear that to record a hologram the two light beams should be mutually coherent. One definition of mutual coherence relates it to the observable visibility of interference fringes formed by two beams that overlap in space [15] , [16] . For continuous wave radiation, the observation of a high contrast fringe pattern is possible if both beams are nearly monochromatic and have identical frequencies. If two coherent light waves (1 and 2) have different frequencies, the fringe pattern that they form moves with the velocity ε =Ω/ K that depends on frequency detuning of the waves, Ω= ω 2 − ω 1 , and spatial frequency K ( K = k 2 − k 1 , k 1 , 2 being the recording beam wave vectors). Taking, for example, blue and green light waves with wavelengths 489 and 500 nm which intersect at an angle of 4°, we get the fringe velocity ε ≈10 8 m s −1 . 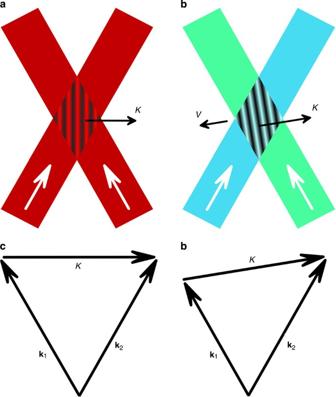Figure 2: Interference of two waves with identical and with different frequencies. Static fringes from two beams with (a) identical frequency spectrum and (b) fringes from beams of different colour that move with the velocityε. The relevant wavevector diagrams (c,d) are shown below the fringe patterns. Figure 2 shows the structure of static fringes for the conventional case of hologram recording (for example, two red beams from continuous wave He–Ne laser) and moving fringes in case of interference of beams of two different colours. Figure 2: Interference of two waves with identical and with different frequencies. Static fringes from two beams with ( a ) identical frequency spectrum and ( b ) fringes from beams of different colour that move with the velocity ε . The relevant wavevector diagrams ( c , d ) are shown below the fringe patterns. Full size image Only the nonlinear processes with instantaneous response can follow the fringes that move with a velocity that is comparable with the velocity of light. Forty years ago the possibility to record a dynamic hologram in a medium with ultrafast response was suggested by Denisijuk [17] . He called this effect ‘holography with intensity waves’. Nowadays, it can be implemented, for example, with two-photon absorption gratings [18] , [19] , which will be discussed in the last section of this paper. The main objective of the present paper is, however, to prove that different colour recording of a holographic grating is possible in any medium, regardless how long is its response time, including media for permanent grating recording. To perform such a recording, we propose to take a snapshot of the moving fringes with a very short exposure time. A simple calculation allows for estimating the distance of fringe displacement Δ ℓ = ετ within the pulse duration τ . If this displacement is smaller or comparable with the fringe spacing Λ=2π/ K the recorded fringe pattern will not be smeared out completely. This gives a hope that femtosecond lasers can be used for holographic grating recording by beams of different colours. The quantitative criteria for getting sufficiently high contrast of the pattern integrated over the pulse duration are derived in the next section. Evaluation of the modulation depth To calculate the modulation depth for a time-integrated fringe pattern as a function of the detuning frequency, we consider the interference of two pulses within the plane waves approximation. The electric field of two waves is with the amplitudes a 1,2 , temporal shape f ( t ), angular frequencies ω 1,2 and wavevectors k 1 , 2 . The pulse duration τ = τ 1 = τ 2 is defined by the FWHM of the intensity profiles I 1,2 ( r , t )=| E 1,2 ( r , t )| 2 . The intensity distribution of the total field in time and space gives then a moving fringe pattern that is represented by Here Ω= ω 2 − ω 1 denotes the frequency detuning and K = k 2 − k 1 denotes the wavevector of the sinusoidal pattern. The pattern moves with the velocity ε =Ω/ K ( K =| K |) along K , and its fringe contrast is given by . In our experiments, this fringe pattern is generated with ultrashort laser pulses ( τ ≈100 fs), and the pulse duration is most often much shorter than the temporal response of the detectors used (digital camera, holographic emulsion and human eye). For single-pulse interference, this yields a time-integrated pattern of energy density per unit area: Note, that ( r ) depends on the temporal shape f 2 ( t ), thus on τ , as well as on the detuning frequency Ω. The modulation depth of the energy distribution ( r ) is analyzed below by assuming three common f ( t ) shapes: rectangular, Gaussian and hyperbolic secant. A rectangular pulse can be expressed by f 2 ( t )=rect[ τ /2, − τ /2] with an intensity that does not change within the total pulse duration τ . This particular shape of I ( t ) simplifies the integration of equation (3) and allows to determine the modulation depth of the energy density pattern as a function of Ω and τ : The two-dimensional plot of is illustrated in Fig. 3a . The largest is reached, naturally, for Ω=0, whatever is the pulse duration τ . The detuning range within which the modulation depth is still high (the width of the central white stripe in Fig. 3a ) depends, however, on pulse duration and increases quite strongly with decreasing τ . (It should be noted that for extremely short pulses (<5 fs) the estimate according equation (5) is senseless because the fringe pattern width in K -direction becomes comparable or smaller than the fringe spacing 2π/ K ). 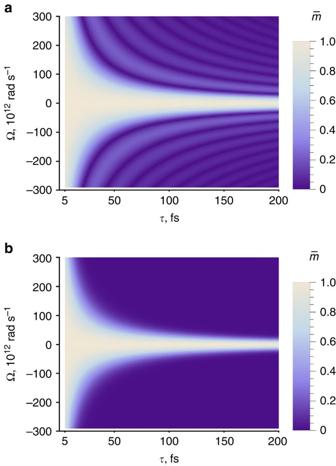Figure 3: Calculated modulation depth averaged over the pulse duration. Modulation depth as a function of frequency detuning Ω and pulse durationτfor (a) rectangular and (b) Gaussian pulse profiles. The interaction of pulses with identical amplitudes is assumed. Figure 3: Calculated modulation depth averaged over the pulse duration. Modulation depth as a function of frequency detuning Ω and pulse duration τ for ( a ) rectangular and ( b ) Gaussian pulse profiles. The interaction of pulses with identical amplitudes is assumed. Full size image For any arbitrary τ (or arbitrary nonzero Ω) the frequency detuning dependence (or pulse length dependence) of shows additional maxima typical to sinc function. The -values of these maxima, as it follows from equation (5), are inversely proportional to the product Ω τ . The sinc-like behaviour vanishes, however, completely under the assumption of a pulse temporal profile with a bell-shaped function, particularly, for a Gaussian profile: or hyperbolic secant prtofile: τ being the FWHM in both cases. Integration of equation (3) then yields: and Figure 3b shows the plot for a Gaussian profile, the plot for a hyperbolic secant profile is qualitatively similar. The characteristic difference between the modulation depth of rectangular, Gaussian and sech pulses is highlighted in Fig. 4 for a fixed detuning of Ω=3 × 10 13 rad s −1 as a double-logarithmic plot. The modulation depth for Gaussian and sech pulses drop as a function of pulse duration in a similar way, while the decay for rectangular pulses is not so strong and is characterized by an oscillatory behaviour. 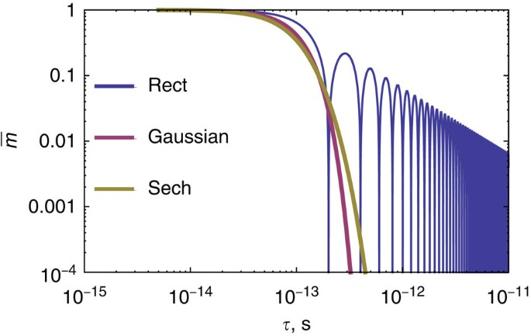Figure 4: Effect of the pulse temporal profile on modulation depth. Comparison of the modulation depth as a function of pulse durationτfor rectangular, Gaussian and hyperbolic secant pulses. A fixed frequency detuning of Ω=3 × 1013rad s−1and equal intensities of two pulses are assumed. Figure 4: Effect of the pulse temporal profile on modulation depth. Comparison of the modulation depth as a function of pulse duration τ for rectangular, Gaussian and hyperbolic secant pulses. A fixed frequency detuning of Ω=3 × 10 13 rad s −1 and equal intensities of two pulses are assumed. Full size image From the viewpoint of our pump–probe experiment described above (Ω≈3 × 10 13 rad s −1 and τ ≈100 fs), it becomes clear that the modulation depth is for a Gaussian pulse (≈0.6 for a rectangular pulse), that is, a fringe pattern with sufficiently high modulation depth is present and is able to cause the recording of a grating. Note, that the generalization to the case of repetitive rate excitation is natural, provided the phase difference of waves in equation (1) does not change from one pulse to the other. The modulation depth is not affected by the number of pulses N because all terms in equation (3) are multiplied to the same number of pulses N . Visualization of interference fringes The visual observation of two-colour beam interference becomes possible by adjusting a small angle between the beams. We note that the fringe velocity ε depends on the fringe spacing Λ, but the condition ετ /Λ≤1 does not impose any restriction to Λ. Thus, the observable fringe contrast should be independent of the angle between the recording beams, and a fringe spacing can be adjusted to be large enough for detection with the naked eye. The schematic representation of the experiment on fringe observation and grating recording is shown in the upper left corner of Fig. 5 . The temporal overlap of pulses from two OPAs on a diffusing white screen is ensured with an optical delay line. With this arrangement, it is possible to observe a fringe pattern on the screen and to register its image. 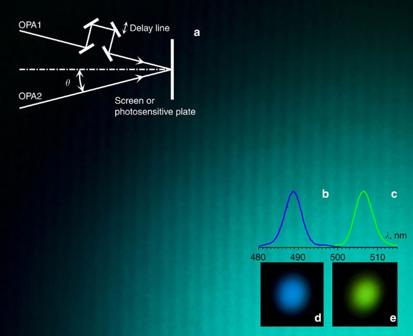Figure 5: Observation of fringe pattern from light beams of different colours. The background image shows a fragment of a fringe pattern from single-pulse light beams withλ=489 and 506 nm. The geometry of fringe observation (a) is shown in upper left corner. The net difference in colours of two beams is clearly seen from measured spectra (b,c), and from near-field distributions (d,e). Figure 5: Observation of fringe pattern from light beams of different colours. The background image shows a fragment of a fringe pattern from single-pulse light beams with λ =489 and 506 nm. The geometry of fringe observation ( a ) is shown in upper left corner. The net difference in colours of two beams is clearly seen from measured spectra ( b , c ), and from near-field distributions ( d , e ). Full size image The very first attempt revealed distinct fringes for quite different wavelengths, that were visible both with single shot and in repetition rate operation mode. An example is shown in Fig. 5 that represents fringes from the beams with 17 nm wavelength detuning. Care is taken to get a uniform transverse intensity distribution in both beams and a good superposition of the spots with nearly equal diameter. The two beams were identically linearly polarized, perpendicularly to the drawing of Fig. 5 . The full angle between the beams was deliberately chosen here to be nearly 0.5° to increase the fringe spacing. The described observation is a purely ‘linear optic’ effect, any kind of nonlinearity is not involved here. The beams interfere only when they are superposed in space and in time. If the observation screen is moved so that the light spots are completely separated, the fringes are no more visible. The fact that a fringe pattern could be observed with naked eye at 1 kHz repetition rate proves that spatial position of fringes remains the same from one pulse to the other, at least during the physiological limit of the human eye response (about 0.04 s). Later this was confirmed when recording the grating with several consecutive pulses: the contrast of the recorded pattern did not deteriorate as compared with single-pulse recording. Such a feature could be expected as one and the same mode-locked Ti–Sapphire laser is initially feeding the two channels in which the recording beams are formed. For both recording beams, the phase of every new pulse in train is not arbitrary and the effective phase difference is preserved from pulse to pulse. It should be underlined, however, that for the case of single-pulse experiment no restrictions are imposed for the light sources that provide two interfering beams: they can be the two completely independent lasers with the outputs of different colour, that in common sense would be considered completely mutually incoherent. The only necessary condition for fringe observation is the spatial and temporal overlap of output ultrashort pulses and their polarization adjustment. In case of repetition rate experiment, there are a few additional requirements—the repetition rates of the two beams should be exactly the same and the coherence time of each beam should be longer than the total time of fringe recording (or fringe observation). As it was mentioned above, these conditions were met in full with the femtosecond laser system used in our experiment. Modulation depth versus wavelength detuning The digitized image like that shown in Fig. 5 allows for evaluating the recorded fringe modulation depth . These measurements were done for a series of fringe patterns that have been taken with the fixed wavelength of one OPA λ 1 =489 nm and variable wavelength of the other OPA. The processing of digitized images and extraction of from the raw data are described in the Methods section. 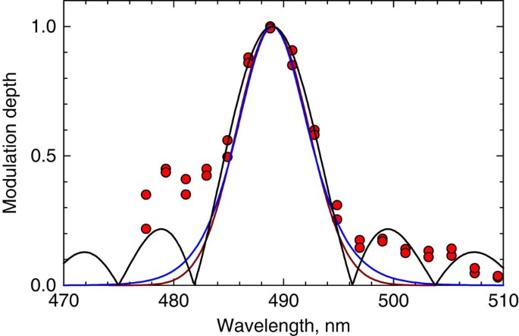Figure 6: Wavelength detuning dependence of the modulation depth. Dots represent the data measured with a fixed wavelength, 488 nm, of one beam and the wavelength variable within the range 475–510 nm for the other beam. Solid lines represent the dependences calculated within the assumption of the rectangular (black), Gaussian (deep red) and hyperbolic secant (blue) temporal envelopes of the interfering pulses. Measurement of fringe contrast Figure 6 shows the detuning dependence of the fringe contrast (dots). The accuracy of estimate is high for small frequency detunings, the uncertainty increases up to ≈30% for largest measured detunings, where the modulation depth becomes small. Figure 6: Wavelength detuning dependence of the modulation depth. Dots represent the data measured with a fixed wavelength, 488 nm, of one beam and the wavelength variable within the range 475–510 nm for the other beam. Solid lines represent the dependences calculated within the assumption of the rectangular (black), Gaussian (deep red) and hyperbolic secant (blue) temporal envelopes of the interfering pulses. Full size image The attempts to fit the measured data with functions calculated in previous section for different intensity profiles of the recording pulses are given by the solid lines: black line represents a sinc(Ω τ /2) dependence for rectangular pulses; the fit yields τ ≈110 fs for the pulse duration. The fitting of functions calculated for Gaussian and hyperbolic secant profiles gives a somewhat smaller pulse duration, about 80 fs. In all cases, however, the estimated values are in reasonable agreement with the directly measured pulse duration of about 100 fs. Grating recording and hologram recording The fringe pattern that can be seen with the eye can also be recorded with a photosensitive medium. Such an imprint of fringes represents a plane wave hologram. They were recorded using conventional silver halid photo emulsions with standard chemical development and subsequent bleaching procedure. For close wavelengths of the two recording beams, the ±2 diffraction orders are clearly seen and the diffraction efficiency in the first order is a few per cent. In the limit of small phase modulations the diffraction efficiency η depends quadratically on fringe contrast (ref. 20 ). Thus the decrease of with the increasing detuning (see Fig. 6 ) should inhibit diffraction. Just this behaviour was observed experimentally. We also registered a hologram in a photoemulsion with an image-bearing beam. The amplitude mask shown in the upper left corner of Fig. 7 was installed in one of the two recording beams (green beam), which is loosely focused. The angle between the recording beams was increased to 4° to ensure that the carrier spatial frequency K of a hologram was larger than the spatial frequency content of the image. 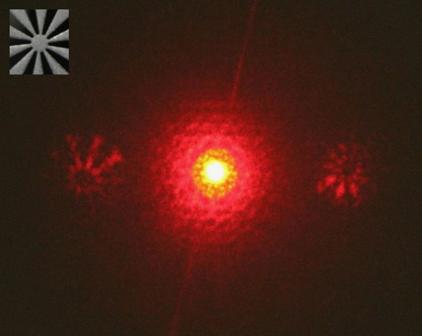Figure 7: Image reconstruction from a hologram recorded with pulses of different colour. Readout with a He–Ne laser of the hologram written by femtosecond pulses with 489 and 501 nm wavelengths. The inset in the upper left corner shows the amplitude mask installed in one of the two beams during recording; grey color marks the areas with zero transmission. Figure 7 shows the reconstructed images, the pseudoscopic on the left side and orthoscopic on the right side from the central spot, which represents the transmitted readout beam from the He–Ne laser. The reconstructed images are quite noisy, however one can recognize unambiguously the original pattern. Figure 7: Image reconstruction from a hologram recorded with pulses of different colour. Readout with a He–Ne laser of the hologram written by femtosecond pulses with 489 and 501 nm wavelengths. The inset in the upper left corner shows the amplitude mask installed in one of the two beams during recording; grey color marks the areas with zero transmission. Full size image It is shown in this paper that the contrast of time average interference pattern of two short light pulses of different colour can be remarkably high at least for frequency detuning |Ω|≤2π/ τ . As it follows from the data of Fig. 6 , the experimental detuning dependence of the modulation depth has rather extended, slightly waving wings. When comparing this result with calculations, one can see that the measured values of for |Ω|≥2π/ τ are obviously larger than that expected for Gaussian and hyperbolic secant temporal profiles. This may point to a pulse shape that is certainly not rectangular but doesn't also have smoothly decaying wings typical for Gaussian and hyperbolic secant functions. The evident asymmetry of dependence can be attributed to the changes of pulse shape and width with the detuning. It should be noted that the problem of effective fringe visibility can be considered not only in time domain, what we did above, but also in the frequency domain. Obviously, a considerable reduction of the pulse duration leads to the broadening of its spectrum. Even a slight spectral overlap of the two pulses may lead to the appearance of a fringe pattern with finite modulation depth. For the case of transform limited pulses, the pulse-bandwidth product is Δ ν × τ = κ . The factor κ is close to unity and depends on the particular pulse shape, for Gaussian pulses κ =2ln(2)/π holds [21] . Therefore, the modulation depth for Gaussian pulses (see equation (8)) can be rewritten in terms of the detuning frequency Ω and the spectral width Δ ω of the pulses (with ν = ω /2π): Taking the experimental conditions λ 1 =489 nm, λ 2 =506 nm and τ =100 fs, we get Ω/Δ ω ≈4.7 for an assumed Gaussian shape, which indicates a small overlap which is due to the extended wings of gaussian pulses as it is shown in right hand side of Fig. 5 . Summarizing, we claim that with 100 fs pulses a recording of holographic grating is possible if the frequencies of two pulses differ up to 4% of the mean optical frequency (larger detunings are allowed for shorter pulses). Of course, when read out with one of the two recording beams, a recorded static hologram can not reproduce the wavelength of the other beam. With some distortions it can reproduce, however, the recorded wavefront. For classical holography the described phenomenon is rather unexpected and obviously new. It can bring new technical solutions for static hologram recording of ultrafast processes, including new variations of Nils Abramson’s light-in-flight holography [2] , [22] . We believe, however, that our result will have a major impact in nonlinear wave mixing and nonlinear spectroscopy. The appearance of transient or permanent grating recorded by two interacting waves may strongly influence the interpretation of pump–probe experiments. Our results described above prove that a direct coupling from such a grating because of self-diffraction affects both the intensity and the spectrum of the probe beam. We limited ourselves in the present paper by consideration of permanent gratings only, as an ultimate case of recording in a material with the infinite storage time. In fact, a vast variety of χ 3 nonlinearities with response times ranging from practically zero to infinity can respond to the described moving fringe pattern, thus bringing particular types of coupling. Apart from the coupling because of self-diffraction, the transient gratings can be revealed through the appearance of higher (non Bragg) orders in case of Raman–Nath diffraction. In media with instantaneous response (other ultimate case compared with described above) the higher orders of diffraction should be upshifted and downshifted in frequency exactly by the frequency difference of the recording waves Ω. Our preliminary experiments with different colour recording of two-photon absorption gratings, that are currently in progress and will be published separately, confirmed the possibility of building such a tunable frequency converter. 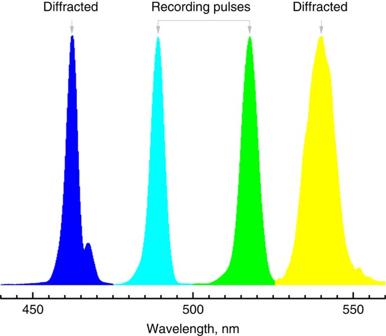Figure 8: Frequency conversion via self-diffraction from a moving dynamic grating. Spectra of the transmitted recording pulses and ±1 diffraction orders. The thin two-photon absorption dynamic grating is recorded in a 200-μm thick sample of LiNbO3by beams that differ by ≈25 nm in wavelength and impinge upon the sample at a full angle of ≈4°. Figure 8 shows an example of up and downconversion to Δ λ ≃ 25 nm with self-diffraction from the moving two-photon absorption grating in a thin sample of LiNbO 3 . The severe fundamental restriction on the diffraction efficiency for amplitude gratings [20] resulted in only 0.01 conversion efficiency in this demonstration experiment. A considerable improvement of efficiency is expected with purely phase moving gratings, profiting from the dominant real part of χ 3 nonlinearities. Figure 8: Frequency conversion via self-diffraction from a moving dynamic grating. Spectra of the transmitted recording pulses and ±1 diffraction orders. The thin two-photon absorption dynamic grating is recorded in a 200-μm thick sample of LiNbO 3 by beams that differ by ≈25 nm in wavelength and impinge upon the sample at a full angle of ≈4°. Full size image A hologram recording in Leith–Upatnieks geometry, with an oblique reference wave, is demonstrated in this article. Taking into account that even in dense media the spatial width of 100 fs pulse is not <10 μm, the reflection gratings and Lippman-type (reflection) holograms can be recorded by counterpropagating light pulses, too. This allows also for considering different applications based on nonlinear backward wave four wave mixing with ultrashort pulses. Dynamic grating techniques have been used successfully in the past for the development of autocorrelation-type measurements of femtosecond pulse duration [3] . With pulses of different colour, this technique can be extended for cross-correlation experiments. The studies of gratings with instantaneous response recorded by pulses of different colours will be profitable for evaluation of a frequency chirp in ultrashort pulses, that is, the short pulse characterization will be another domain to apply the described phenomenon. Finally, this work will trigger new attempts to reconsider the definition of coherence for pulsed radiation. In particular, the question will be discussed—can the blue pulse and green pulse from two different lasers be considered mutually coherent? Laser system and optical set-up The femtosecond laser system used in the experiment consists of several separate devices in chain; Fig. 9 shows it schematically. A mode-locked Ti 3+ :Al 2 O 3 oscillator generates the initial train of femtosecond pulses with a spectrum centred at wavelength λ =802 nm. Chirped-pulse amplification is used to reach a maximum pulse energy of (4±0.1) mJ at a repetition rate of 1 kHz. By tuning the compressor grating (C), the pulse duration is adjusted to (100±10) fs, as determined by interferometric auto correlation (Gaussian shape approximation, A.P.E., model: Pulse Check PD 15 ps). The pulses then enter two OPAs (OPA (1) and OPA (2)) with input pulse energies of ≈2.5 mJ and ≈1.5 mJ, respectively, after passing a telescope and a 65:35 beam splitter. 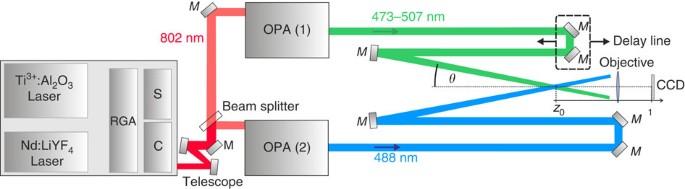Figure 9: Experimental set-up. Femtosecond pulses from a Ti3+:Al2O3laser are stretched (S) to the picosecond length, regeneratively amplified (RGA) using a Ti3+:Al2O3that is pumped by a Q-switched Nd:LiYF4laser (λ=527 nm) and compressed (C) to pulses with 100±10 fs duration and 4 mJ energy (Coherent Inc., LIBRA-HE). The amplified fematosecond pulses serve as a pump for two optical parametric amplifiers (OPA, Coherent Inc., OPerA Solo) to generate femtosecond-laser pulses in the blue–green spectral range via sum-frequency conversion. The optical path lengths of the frequency-detuned pulses is adjusted by a delay line. The pulses are superimposed at a small angle in air, so that the fringe pattern could be imaged onto a screen with lens L. Figure 9: Experimental set-up. Femtosecond pulses from a Ti 3+ :Al 2 O 3 laser are stretched (S) to the picosecond length, regeneratively amplified (RGA) using a Ti 3+ :Al 2 O 3 that is pumped by a Q-switched Nd:LiYF 4 laser ( λ =527 nm) and compressed (C) to pulses with 100±10 fs duration and 4 mJ energy (Coherent Inc., LIBRA-HE). The amplified fematosecond pulses serve as a pump for two optical parametric amplifiers (OPA, Coherent Inc., OPerA Solo) to generate femtosecond-laser pulses in the blue–green spectral range via sum-frequency conversion. The optical path lengths of the frequency-detuned pulses is adjusted by a delay line. The pulses are superimposed at a small angle in air, so that the fringe pattern could be imaged onto a screen with lens L. Full size image Both OPAs use a supercontinuum source of Al 2 O 3 for the signal generation, and a double-stage parametric amplifier scheme (non-collinear and collinear optical amplifier) for signal amplification. Pulses in the blue–green spectral range (470–520 nm) are obtained within a sum-frequency mixing scheme. At the OPA output, pulse energies up to 150 μJ are available with pulse durations <100 fs. The optical paths of the frequency-detuned pulses are matched by using an optical delay line in one of the beams. For the generation of a fringe pattern, the pulses are superimposed at an angle of a few degrees in air at position z 0 . The pattern is imaged by a lens (magnification factor: × 50) onto a screen and grabbed by a digital camera. A metallic mask was placed in one of the two beam paths to demonstrate holographic image recording with a holographic emulsion (Slavich, PFG-03M) at z 0 . The exposed films were chemically processed and reconstructed by a He–Ne laser. Pump–probe experiment The transmittance of a 200-μm thick y -cut sample of a nominally undoped LiNbO 3 crystal was tested with the an ≈100-fs probe pulse in presence of pump pulse with the same duration. The average intensities of the pump and probe pulses were 5.6 PW cm −2 and 0.7 TW cm −2 , respectively. Both pulses, probe and pump, are identically and linearly polarized along the crystal c -axis, they impinge upon the sample in a plane normal to this axis, to avoid a photorefractive grating formation. The spectrum of the pump pulse is fixed at 490 nm while the wavelength of the probe pulse is tunable. The 100 μm beam waist of the probe pulse is roughly 1.5 times smaller than that of the pump pulse. For the wavelength range used in the experiment, even with relatively small full angle between the beams ( ≃ 2.5°) at least 10 interference fringes are expected within the area where two beams overlap. No cumulation effects have been observed; the measurements are done either within a single short pulse or by averaging the data of consecutive 10 pulses. Measurements of fringe contrast To extract the data on fringe contrast from the digitized image of interference pattern, two problems must be solved. First, one needs to be sure that the recording device (digital camera in our case) works within the intensity range where its response to the intensity is linear. Second, for any particular pattern to be processed it is necessary to know the intensity ratio of two interfering beams. Initially the intensity ratio of two waves with identical frequencies was adjusted to be 1:1, it was, however, changing when the frequency of one wave was tuned. Thus, there are two reasons for decreasing the measured modulation depth with the detuning frequency, one is related to variation of the intensity ratio and the other is related to the fringe pattern motion. Whole-measurement procedure was as follows. At first, the two beams were superposed in a best way on a white screen. Then, the digital camera with the removed lens was installed so that its sensitive matrix appeared in a plane of white screen, just in the maximum of the intensity spatial distribution. The matrix dimension, 17 × 22 mm 2 , was roughly 10 times smaller than the FWHM of the interfering beams. The linearity of camera response was ensured by appropriate choice of neutral density filters. To find the intensity ratio of the recording waves, the three measurements were done for every new frequency detuning: the measurements of each interfering beam separately and the measurement of fringes from two superposed beams. Figure 6 shows the recalculated detuning dependence of the fringe contrast (dots), which is due to the fringe motion only. How to cite this article: Odoulov, S. et al . Interference and holography with femtosecond laser pulses of different colours. Nat. Commun. 6:5866 doi: 10.1038/ncomms6866 (2015).